Probing charge scattering mechanisms in suspended graphene by varying its dielectric environment Graphene with high carrier mobility μ is required both for graphene-based electronic devices and for the investigation of the fundamental properties of Dirac fermions. An attractive approach to increase the mobility is to place graphene in an environment with high static dielectric constant κ that would screen the electric field due to the charged impurities present near graphene's surface. Here we investigate the effect of the dielectric environment of graphene and study electrical transport in multi-terminal graphene devices suspended in liquids with κ ranging from 1.9 to 33. For non-polar liquids ( κ <5), we observe a rapid increase of μ ( κ ), with room-temperature mobility reaching ~60,000 cm 2 Vs −1 for devices in anisole ( κ =4.3). We associate this trend with dielectric screening of charged impurities adsorbed on graphene. We observe much lower mobility μ ~20,000 cm 2 Vs −1 for devices in polar liquids ( κ ≥18) and explain it by additional scattering caused by ions present in such liquids. Charge scattering in graphene has been the subject of intense investigation ever since its discovery [1] . Clean graphene specimens with high carrier mobility μ are required both to probe the properties of graphene's Dirac fermions [2] and to realize a plethora of proposed graphene-based electronic devices [3] , [4] . It is now largely accepted that the mobility-limiting factor in graphene is the Coulomb scattering off of charged impurities that reside either on graphene or in the underlying substrate [5] . This is true both for traditional graphene devices on SiO 2 substrates [5] and possibly for the recently reported high-mobility suspended [6] , [7] and supported [8] devices. An attractive approach to reduce such scattering is to place graphene in an environment with a high static dielectric constant κ that would effectively screen the electric field due to the impurities [9] , [10] , [11] , [12] . However, experiments so far report only a modest effect of high- κ environments on mobility [13] , [14] . While one study initially reported a large value of mobility for graphene covered by a high- κ medium [15] , a later work by the same group showed that those claims were unfounded and resulted from an error in the measurement process [16] . Hence, despite significant progress in understanding the electron transport in graphene, the role of graphene's dielectric environment in screening the scattering has not been elucidated yet. Here we investigate the effect of the dielectric environment of graphene by studying electrical transport in multi-terminal graphene devices that are suspended in liquids with a static dielectric constant κ ranging from 1.9 to 33. For non-polar liquids ( κ< 5), we observe a rapid increase of μ with κ and report a room-temperature mobility as large as ~60,000 cm 2 Vs −1 for graphene devices in anisole ( κ =4.3), while in polar liquids ( κ ≥18) we observe a decrease in μ to values measured in conventional graphene field-effect transistors on SiO 2 . We demonstrate that non-polar liquids enhance mobility by screening charged impurities adsorbed on graphene, while charged ions in polar liquids cause the observed mobility suppression. Furthermore, using molecular dynamics simulation, we establish that scattering by out-of-plane flexural phonons, a dominant scattering mechanism in suspended graphene in vacuum at room temperature (RT) [17] , is suppressed by the presence of liquids. We expect that our findings may provide avenues to control and reduce carrier scattering in future graphene-based electronic devices. Sample fabrication and measurements To vary the dielectric constant of graphene's environment controllably, we fabricated nine large (2–4 μm by 8–10 μm) multi-probe graphene devices that are suspended in liquids with the dielectric constant κ varying from ~1.9 to ~33 ( Fig. 1 ). The liquids are non-polar solvents—hexane ( κ =1.9), toluene (2.3), anisole (4.3), as well as polar liquids—isopropanol (18), ethanol (25) and methanol (33). Large leakage currents prevented us from measuring the devices in solvents with higher κ , such as water ( κ =79). We expect that changes of κ should significantly affect electrical transport in suspended devices, as both sides of the graphene sheet are exposed to the high- κ medium and as substrate-induced scattering is effectively eliminated, leaving only scattering from charged impurities on the surface of graphene. During the course of the experiments, we study the electric transport parameters—conductivity ( σ ), Hall carrier mobility ( μ ) at n =5×10 11 cm −2 and effective capacitance ( C g ) using the same device suspended in different liquids at RT and under ambient conditions. To ensure that no additional scatterers are adsorbed onto the device between the measurements, we never dried the devices during the experiment (see Methods ). 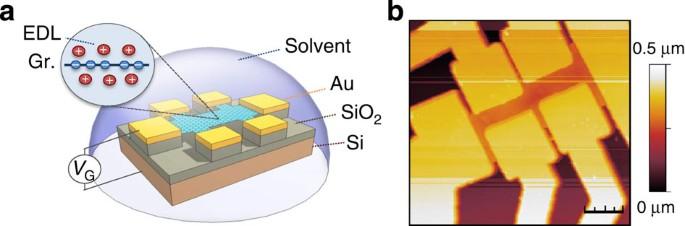Figure 1: Multi-terminal graphene device suspended in liquids with varying dielectric constant. (a) Device schematics: gold electrodes support a graphene sheet ~200 nm above the SiO2/Si substrate; liquid surrounds the entire device. When a potential is applied between the graphene and the gate electrode, an ionic electric double layer (EDL) forms next to the graphene (Gr.). (b) The suspended graphene device dried and imaged in air using an atomic force microscope after the completion of measurements. Imaging confirms that the device remained suspended during the course of the experiments, rather than collapsed onto the substrate. The specimen shown is smaller than the typical devices used in the experiments. The scale bar is 2 μm. Figure 1: Multi-terminal graphene device suspended in liquids with varying dielectric constant. ( a ) Device schematics: gold electrodes support a graphene sheet ~200 nm above the SiO 2 /Si substrate; liquid surrounds the entire device. When a potential is applied between the graphene and the gate electrode, an ionic electric double layer (EDL) forms next to the graphene (Gr.). ( b ) The suspended graphene device dried and imaged in air using an atomic force microscope after the completion of measurements. Imaging confirms that the device remained suspended during the course of the experiments, rather than collapsed onto the substrate. The specimen shown is smaller than the typical devices used in the experiments. The scale bar is 2 μm. Full size image Transport in graphene suspended in non-polar solvents Polar and non-polar liquids have a very different effect on electrical transport in suspended graphene ( Fig. 2a ). In non-polar liquids, we observe an increase of μ ( =σ/ne at n =5×10 11 cm −2 ) with κ for every measured device ( Fig. 2b ). In a representative device (Device #1), the mobility increases from μ ~29,000 cm 2 Vs −1 in hexane ( κ =1.9) to a large value μ ~45,000 cm 2 Vs −1 in anisole ( κ =4.3), more than twice the value for the same device on a substrate ( Fig. 2a , dashed curve). In a different device (Device #2), the mobility in anisole reached ~60,000 cm 2 Vs −1 ( Supplementary Fig. S1 ). To the best of our knowledge, this is the highest reported mobility for a graphene device at RT and close to the highest RT mobility seen in any semiconducting material [18] (while higher mobility values are reported in a very recent paper [19] , these values are measured at a lower temperature ~250 K and at a lower carrier density). In general, the mobility measured for any device in anisole is always approximately 100–250% higher than the mobility for the same device either measured in hexane or in air before suspension. The devices are stable over days of measurements and exhibit changes in μ <10% on cycling multiple times through various solvents ( Supplementary Fig. S2 ). At the same time, despite large changes in μ , the minimal conductivity σ min is not affected by graphene's dielectric environment ( Fig. 2a , inset). Qualitatively, the behaviour observed in non-polar liquids is consistent with Coulomb scattering due to charged impurities/residues adsorbed on the graphene surface being the dominant scattering mechanism. Indeed, the potential due to such impurities is expected to be strongly screened in solvents with higher κ (refs 9 , 10 , 11 , 12 ). 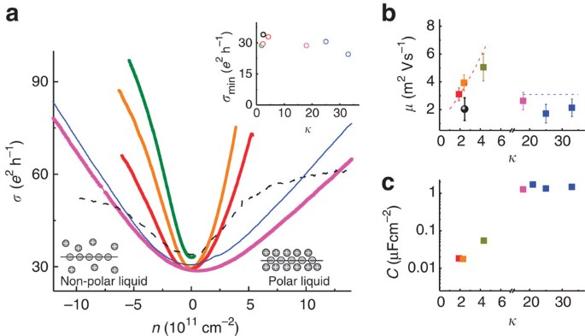Figure 2: Effect of the dielectric environment on the transport properties of a suspended graphene device. (a) The conductivityσas a function of carrier densitynfor representative suspended device #1 in different liquids; hexane (red solid line), toluene (orange), anisole (green), isopropanol (magenta) and ethanol (blue). For comparison, the black dashed line representsσ(n)of the same device #1 supported on SiO2and not covered by any liquid. (That data were obtained before the substrate under the device was etched away during the fabrication stage). Note thatσ(n)is sublinear when the same device is measured in air before suspension and becomes linear after suspension in liquids. The inset (top): the minimal conductivityσminof the same device versus the dielectric constantκof the liquid. (b) The mobilityμatn=5×1011cm−2, averaged over nine measured suspended graphene devices as a function ofκof the liquid (not every device was measured in every liquid). The black circle is the average mobility measured for eighteen reference graphene devices supported on SiO2and not covered by any liquid. The red dashed line is the estimated mobility limited by Coulomb scattering from charged impurities adsorbed on graphene at a concentrationnimp=1×1011cm−2. The blue dashed line is a model that includes ion-induced Coulomb scattering, charged-impurity scattering with the samenimpand withκfixed atκ=6. (c) The measured effective gate capacitanceCGfor the device#1 versusκof the liquid surrounding it. Figure 2: Effect of the dielectric environment on the transport properties of a suspended graphene device. ( a ) The conductivity σ as a function of carrier density n for representative suspended device #1 in different liquids; hexane (red solid line), toluene (orange), anisole (green), isopropanol (magenta) and ethanol (blue). For comparison, the black dashed line represents σ(n) of the same device #1 supported on SiO 2 and not covered by any liquid. (That data were obtained before the substrate under the device was etched away during the fabrication stage). Note that σ(n) is sublinear when the same device is measured in air before suspension and becomes linear after suspension in liquids. The inset (top): the minimal conductivity σ min of the same device versus the dielectric constant κ of the liquid. ( b ) The mobility μ at n =5×10 11 cm −2 , averaged over nine measured suspended graphene devices as a function of κ of the liquid (not every device was measured in every liquid). The black circle is the average mobility measured for eighteen reference graphene devices supported on SiO 2 and not covered by any liquid. The red dashed line is the estimated mobility limited by Coulomb scattering from charged impurities adsorbed on graphene at a concentration n imp =1×10 11 cm −2 . The blue dashed line is a model that includes ion-induced Coulomb scattering, charged-impurity scattering with the same n imp and with κ fixed at κ= 6. ( c ) The measured effective gate capacitance C G for the device#1 versus κ of the liquid surrounding it. Full size image Transport in graphene suspended in polar solvents For the graphene devices suspended in polar solvents with κ ≥ 18, we observed significantly lower mobility values, comparable with or lower than for the same device in air ( Fig. 2a,b ), measured before suspension. This reverses the trend of mobility increasing with κ observed for the devices in non-polar solvents. We propose that the lowering of the mobility indicates an additional scattering mechanism that dominates in polar liquids—Coulomb scattering of graphene charge carriers by charged ions that are present in polar liquids. Indeed, charged ions, likely the results of contamination with ambient water vapour or trace impurities, are always present in liquids at ambient conditions, with concentrations greater for polar than in non-polar liquids [20] . To quantify the presence and the distribution of the ions, we examine the variation of the device capacitance C g in different liquids. While C g measured in non-polar solvents is close to the values measured in air for devices on the SiO 2 (300 nm)/Si substrates, C g ~120 aFμm −2 , the capacitance reaches values up to >1×10 4 aFμm −2 in polar solvents, such as in ethanol ( Fig. 2c ). We interpret the increase of capacitance as a simple consequence of the so-called electrolyte gating [21] (more details in Methods and Supplementary Fig. S3 ). As the back-gate electrode is in contact with the liquid, the electrical potential of the bulk liquid acquires values that are a fraction of the back-gate voltage V g and an ionic electrical double layer (EDL) with a characteristic thickness d (Debye length), forms next to the graphene ( Fig. 1a ). The formation of an EDL results in a strong electric field at the graphene–liquid interface, which in turn results in a large apparent back-gate capacitance [22] . Using the Gouy–Chapman–Stern model, we estimate d~ 2 ɛ 0 κ/C g , and obtain d ≥ 140 nm for non-polar and d ≤ 12 nm for polar solvents (details in Supplementary Methods ). Therefore, in polar solvents, the ions are in close proximity to the graphene and can contribute to Coulomb scattering ( Fig. 2a , bottom inset). Transport in graphene suspended in salted non-polar solvent To confirm the role of the charged ions in limiting the mobility of graphene, we also studied the same suspended graphene device#1 in a non-polar solvent, anisole, into which we artificially introduced charged ions by adding tetrabutylammonium tetraphenylborate (TBATPhB) salt in concentrations varying from 0 to 80 mM ( Fig. 3a ). As expected, the increased ionic concentration resulted in an increase in capacitance ( Fig. 3b ) and a decrease in mobility ( Fig. 3c ), reflecting the increased scattering and higher electric fields due to the ions being on average closer to the graphene at a higher salt concentration. 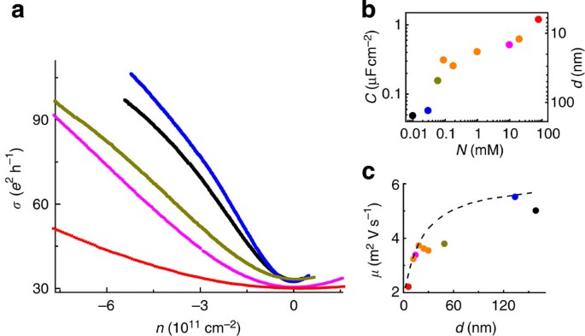Figure 3: Effect of the ions in the liquid on electrical transport of suspended graphene device. (a) Conductivityσ(n)of device #1 measured in anisole salted with TBATPhB for different concentrations of TBATPhB,N=0 μM (black line), 30 μM (blue), 60 μM (green), 10 mM (magenta) and 80 mM (red). (b) CapacitanceCgand the average thickness of the EDLdestimated fromCgversus salt concentration for the same device. (c) The mobilityμversus the EDL thicknessd. The dashed line is the expectation of the Coulomb scattering model that includes the scattering by the impurities with the concentrationnimp~1×1011cm−2attached to the graphene surface and the contribution due to ions in solution. Figure 3: Effect of the ions in the liquid on electrical transport of suspended graphene device. ( a ) Conductivity σ(n) of device #1 measured in anisole salted with TBATPhB for different concentrations of TBATPhB, N =0 μM (black line), 30 μM (blue), 60 μM (green), 10 mM (magenta) and 80 mM (red). ( b ) Capacitance C g and the average thickness of the EDL d estimated from C g versus salt concentration for the same device. ( c ) The mobility μ versus the EDL thickness d . The dashed line is the expectation of the Coulomb scattering model that includes the scattering by the impurities with the concentration n imp ~1×10 11 cm −2 attached to the graphene surface and the contribution due to ions in solution. Full size image Transport in graphene supported on SiO 2 substrate We compared the μ ( κ ) dependence observed for suspended devices with μ ( κ ) measured for devices supported on a SiO 2 substrate and covered with liquid. We prepared four different supported devices with the Hall bar geometry that had similar dimensions compared to the devices discussed above, and were fabricated using the same techniques except for the final etching step. In addition, we studied two supported devices that were thermally annealed in forming gas (300 °C for 2 h in 1:4 H 2 /Ar gas at 2.3 Torr) to remove the photoresist residues [23] , [24] , before depositing liquids onto graphene. Similar to the previous report [14] , we observed only a weak dependence of mobility on κ in these supported devices. In addition, the measured mobility values were significantly lower compared with the mobility observed for suspended devices ( Supplementary Fig. S4 ). We speculate that this weak μ ( κ ) dependence is caused by two reasons. First, only one side of a supported graphene sheet is exposed to the liquid. In that case, the effective dielectric constant of graphene's environment, κ eff =( κ Liquid + κ SiO2 )/2, has weaker dependence on the dielectric constant of the liquid compared with a suspended device. Second, even after annealing in forming gas, the surface of a supported device is likely to be contaminated with fabrication residues, which should also result in a lower effective dielectric constant, and hence lower mobility values. Our data for suspended graphene devices feature two main trends: a large enhancement of mobility with κ for devices in non-polar solvents, and relatively low values of mobility for devices in polar solvents. To describe this behaviour semiquantitatively, we use a model that includes only two sources of scattering: Coulomb scattering from charged impurities with density n imp —likely the fabrication residues [24] , [25] —located on the graphene sheet [26] , and Coulomb scattering from ions in solution belonging to the EDL (we discuss possible contribution of other scattering mechanisms later). As electric fields are absent in the bulk of the solution, the areal density of these ions n ion has to be equal and opposite in polarity to the carrier density n in graphene. The spatial distribution of ions away from graphene is derived from the Gouy–Chapman–Stern model [22] , while the average thickness of the EDL d is obtained from the C g measurements ( Supplementary Methods ). Both types of scattering mechanisms are screened by the dielectric surrounding the graphene. The scattering rate due to each mechanism is calculated using the semiclassical theory developed by Adam and Das Sarma [26] , and finally Matthiessen's rule is used to get the total rate (See Methods ). In non-polar solvents, where the ionic concentration is negligible (<10 μM), we assume that the Coulomb scattering from charged impurities is the only scattering mechanism at work. We fit our data considering n imp as the only variable parameter ( Fig. 2b , red dashed line) and obtain a good fit with a realistic n imp ~1×10 11 cm −2 . As expected, this value is lower than the values found for the supported graphene and higher than that for suspended graphene in high vacuum [26] . Remarkably, for the case of TBATPhB in anisole, where both scattering mechanism are in function, a reasonable fit is obtained using the same n imp and no adjustable parameters (dashed line in Fig. 3c ). On the other hand, for polar solvents, such as ethanol, the model predicts almost complete suppression of both scattering mechanisms due to screening and a very high mobility μ >30 m 2 Vs −1 , much larger than observed in the experiment. We resolve this conundrum by noting that at the EDL, the bulk dielectric constant of a liquid ( κ =25 in case of ethanol) can be suppressed by an order of magnitude due to the preferential orientation of polar molecules next to the metal interface [27] , [28] . While to our knowledge there is no detailed theory to describe κ of the EDL, we note that the μ -values measured for polar solvents are consistent with the effective κ ~6, which is close to κ measured for the interfacial layer of water [28] ( Fig. 2b , blue dashed line). We also note that Coulomb scattering due to the dipole moments of polar molecules [29] can be an additional scattering mechanism leading to a decrease in mobility in polar solvents. It is instructive to consider one interesting aspect of the ion-induced carrier scattering. As n ions =− n , the semiclassical estimate for conductivity limited by ion and impurity Coulomb scattering [8] at first glance yields σ ( n )~ n /| n imp + n ion |~ n /| n ion |~const for high carrier densities ( n >> n imp ). This is different from the roughly linear dependence observed in experiments ( Figs 2a and 3a ). However, this contradiction can be resolved by remembering that the thickness d of the EDL also decreases with n ( Fig. 3b ), and hence a weaker scattering is expected at lower carrier densities. Precise modelling of the σ(n) due to ion-induced scattering is outside the scope of this article and awaits an appropriate theoretical model. However, the dependence n ion =− n means that the surface density of ions in the EDL is exactly zero when graphene is at its charge neutrality point, n =0. Thus, we expect that the electron transport in graphene at the charge neutrality point is unaffected by the ion-induced scattering, and that the scattering is dominated by surface-bound impurities. This prediction is consistent with the observed behaviour of minimum conductivity σ min of our devices, which fluctuates <10% in the same device across the entire range of polar and non-polar solvents ( Fig. 2a , Inset). Indeed, a self-consistent theory [11] predicts the variation in σ min <10% in the range of κ =2 to 33 assuming a constant n imp . Similar nearly constant σ min was also observed in an experiment where κ of graphene's environment was adjusted, albeit in much smaller range [10] . We note that the minimum conductivity of our devices ( σ min ~30 e 2 h −1 for the device shown in Fig. 2a ) is significantly larger compared with typically reported values [30] . We speculate that this is a consequence of the unintentional electrode doping of our devices [31] , [32] , [33] (see Methods and Supplementary Methods ). Finally, we analyse the implicit assumption of our model that the Coulomb scattering is the dominant scattering mechanism in our devices. First, disorder of graphene (that is, dislocations in the lattice) can cause significant short-range scattering in high-mobility suspended devices [13] , [34] , [35] . However, it has been proposed theoretically [36] , [37] and recently confirmed experimentally [13] that the strength of such scattering should increase with increasing dielectric constant of graphene environment. The opposite trends are observed in our experiments. Second, recent experiments reported strong scattering of charge carriers in graphene by out-of-plane (flexural) phonons for suspended graphene in vacuum [12] . The values of the mobility observed here are significantly larger than the mobility limitation μ <30,000 cm 2 Vs −1 due to scattering on flexural phonons [17] . To resolve this seeming contradiction, we performed molecular dynamics simulations of graphene sheets suspended in either hexane, toluene or in vacuum at RT. We find that the interaction of molecules of the liquid with graphene suppresses the amplitude of the phonons by ~50% ( Fig. 4 ). We also verified computationally that this suppression is equivalent to an effective increase of the bending rigidity [38] of graphene k from a free-space value ~1.3 eV in vacuum to ~3.6 eV for graphene suspended in hexane or toluene ( Supplementary Fig. 5a,b and discussed in the Supplementary Methods ). This, in turn, translates to a mobility limitation due to phonons ( μ lim ~const× k 2 , from ref. 17 ) of ~230,000 cm 2 Vs −1 . As this is significantly larger than the values of μ in our devices, we conclude that the scattering by the out-of-plane acoustic phonon is insignificant in our experiments due to the suppression of these phonons in the presence of a liquid. 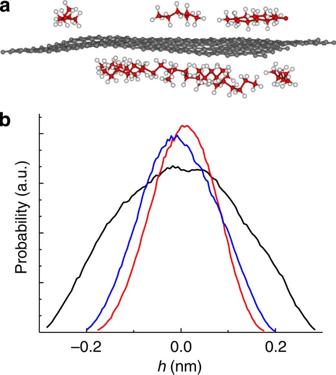Figure 4: Molecular dynamics simulations of flexural phonons (ripples) in suspended graphene in liquids and in vacuum at room temperature. (a) A snapshot from the simulation of graphene in hexane (not all the hexane molecules are shown). (b) Probability distribution for heights (h) of a graphene sheet suspended in hexane (blue line), toluene (red) and in vacuum (black). Note that the ripples are significantly suppressed in non-polar solvents. (a.u., arbitrary unit). Figure 4: Molecular dynamics simulations of flexural phonons (ripples) in suspended graphene in liquids and in vacuum at room temperature. ( a ) A snapshot from the simulation of graphene in hexane (not all the hexane molecules are shown). ( b ) Probability distribution for heights ( h ) of a graphene sheet suspended in hexane (blue line), toluene (red) and in vacuum (black). Note that the ripples are significantly suppressed in non-polar solvents. (a.u., arbitrary unit). Full size image Our observations may have several important consequences. First, the demonstrated increase of mobility in non-polar liquids with high κ may provide a viable approach towards engineering of high-mobility graphene devices that operate at RT. Second, we resolve the apparent contradiction between the previously reported experimental data for graphene in high- κ environment [13] , [14] and the Coulomb scattering theory [9] , [10] , [11] , [12] . Third, the demonstrated sensitivity of electron transport in graphene to the presence of ions in solution may lead to a new paradigm of electrochemical sensors and biosensors [39] . Finally, we expect that the rich physics of ion–electron interaction encountered here may stimulate the development of a theory describing electron transport of graphene in ionic solutions. Fabrication of suspended graphene devices The suspended graphene devices in liquid ( Fig. 1a ) are prepared following previous work [6] . Briefly, graphene is obtained by micromechanical exfoliation, gold/chrome electrodes are fabricated via electron beam lithography followed by metal evaporation, and the sacrificial SiO 2 is removed via etching in hydrofluoric acid ( Supplementary Methods ). The monolayer graphene was confirmed by micro-Raman spectroscopy [40] . Crucially, the devices are never dried after etching to avoid the collapse of graphene onto the substrate due to surface tension of the drying liquid [6] . Instead, the etchant was slowly replaced by deionized water and then by the high- κ liquid under study. A total of nine suspended devices in different liquids were studied. In control experiments, we also examined 18 graphene devices supported on SiO 2 in air, four supported devices on SiO 2 with liquids on top of them and two thermally annealed supported graphene devices with liquids on top of them ( Supplementary Table S1 ). Electrical transport measurements These measurements are performed under ambient conditions at RT. We use standard four-probe measurements at low magnetic field B (0–46 mT) to determine the Hall resistivity ρ x y , the carrier density n = B/eρ xy , the gate capacitance C g = edn/dV G ( V G is the gate voltage) and the carrier mobility μ ( n max )=( L / W) ×1/( R xx ne ) at the maximum density n max =5×10 11 cm −2 accessible in our devices, where L is the length and W is the width of the channel ( Supplementary Fig. S6 and Supplementary Methods ). Unlike the suspended devices studied by others [6] , [7] , our specimens were never current-annealed. To eliminate any potential errors in measuring the conductivity that could stem from the hysteresis in ρ ( V G ) curves ( Supplementary Fig. S7 ), we have used very low sweeping rate for the gate voltage (~5 mV s −1 for polar solvents). Moreover, the same gate voltage sweeping direction was maintained when recording the ρ xx ( V G ) and ρ xy ( V G ) curves. Uncertainty in determining σ min and μ Only the devices with reasonably small area can successfully survive the suspension step, while larger device can rip or collapse onto a substrate [6] . Therefore, we intentionally have chosen the graphene flakes that are approximately 8–12 μm in length and approximately 2–4 μm in width and are very close to a rectangular shape to fabricate into the devices. The computer-aided design of a typical device is presented in Supplementary Fig. S8a . To determine the uncertainty in the measurements of conductivity that can arise as a result of the inaccuracies associated with the determination of the geometrical factor L/W , we have conducted control experiments using graphene devices of different geometrical factors ( Supplementary Figs S8 and S9 and Supplementary Methods ). We estimate the uncertainty in mobility to be ~20%. At the same time, unintentional electrode doping [31] , [32] , [33] due to closely spaced electrodes can cause significant inaccuracies up to a factor of ~2 in the determination of the minimum conductivity. Electrolyte gating of graphene devices In a majority of the experiments where electrolyte gating is used, a slightly different approach is used. A separate platinum electrode that is not connected to the device is placed into solution and the potential of the liquid is adjusted by applying voltage to that electrode [21] . We have confirmed that this approach is also applicable in our experiments. We placed a platinum needle into the liquid ~1 mm above the surface of graphene suspended in polar solvents and recorded the change in the carrier density with respect to the voltage applied to the electrode. The gate capacitance is similar to the capacitance measured when back-gate biasing is used ( Supplementary Fig. S3b ). Measurements of the voltage drop across EDL In analysing the transport data, it is important to know the part of the voltage applied to the back-gate electrode that falls across the EDL. This drop is the difference between the potential in the bulk of the liquid, which is denoted by V L , and graphene, which is kept at zero potential. To estimate the potential of the bulk of the liquid V L as a function of the potential of the back-gate electrode V G , we placed a separate platinum electrode into the liquid and adjusted its potential until no current flows between it and the liquid. We then assumed that at that point the electrode is at the potential of the liquid V L . We repeated the procedure for different values of V G and recorded V L ( V G ) curve. For all polar liquids used in the experiments, we found that V L ~0.4 V G . As expected, approximately half of V G falls across gate electrode/liquid interface and another half across liquid/graphene interface. Scattering due to impurities adsorbed on graphene We assume that the carrier scattering in our devices is dominated by (1) scattering by the charged impurities—possibly ambient hydrocarbon molecules or residues of the Poly(methyl methacrylate) (PMMA) resist used during the fabrication—adsorbed on the surface of graphene with surface density n imp and (2) Coulomb scattering by charged ions present in solution. To calculate the mobility limitation due to the first mechanism, we use the semiclassical theory developed by Adam and Das Sarma. [26] : Here s is the distance between the charged impurity and graphene, a =4 π 1/2 sn 1/2 , r s is the effective fine structure constant and κ is the dielectric constant of the liquid surrounding graphene. Following the previous work, we assumed s= 0 for the impurities adsorbed on graphene [26] . We have found that at n imp ~1×10 11 cm −2 , the model provides a reasonable fit to our experimental data ( Fig. 2b , dashed line). The predicted and observed increase of mobility with κ originates from the increased screening of the electric field of the impurities by the dielectric environment surrounding graphene. Mobility due to scattering by the ions in solution We now turn to the calculation of the Coulomb scattering due to the charged ions in solution next to the graphene sheet. First, consider one thin layer of solution that is parallel to graphene, at a distance x away from it, and of thickness dx . Using the Gouy–Chapman–Stern model, we obtain the areal density of ions inside this layer ( Supplementary Methods ): The factor 2 appears because both surfaces of the graphene are exposed to the liquid. If only the ions inside this layer were contributing to the scattering of charge carriers in graphene, we can calculate the mobility limitation due to scattering by only these ions using equation (1). The total contribution of all the ions surrounding the graphene can be estimated by summing up the contribution from each layer via Matthiesen's rule, Finally, we once again use Matthiesen's rule to calculate the mobility limitation due to the scattering both by the ions in solution and by the impurities adsorbed on graphene, The result of this modelling is shown as a dashed line in Fig. 3c . The density of the impurities adsorbed on graphene used in calculating μ imp was extracted from the measurements of the same device in non-polar solvents. How to cite this article: Newaz, A. K. M. et al . Probing charge scattering mechanisms in suspended graphene by varying its dielectric environment. Nat. Commun. 3:734 doi: 10.1038/ncomms1740 (2012).